Methane formation driven by light and heat prior to the origin of life and beyond 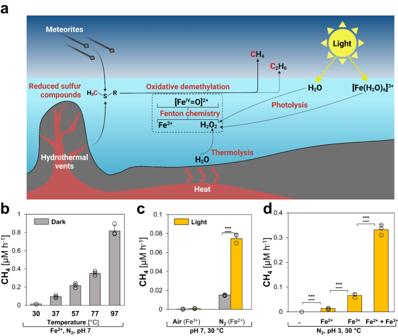Fig. 1: Heat and light drive CH4formation under abiotic conditions. aReduced, methylated S-/N-compounds are formed abiotically in hydrothermal vents or transported to Earth by carbonaceous meteorites. Under anoxic conditions, H2O2is formed by thermolysis and photolysis of water and [Fe(H2O)6]3+complexes, reacting with dissolved ferrous iron (Fe2+) to hydroxyl radicals (∙OH) and [FeIV= O]2+compounds that drive the oxidative demethylation of methylated S-/N-compounds, thereby facilitating CH4and C2H6formation.bThermolysis: CH4is formed from DMSO under high temperatures.cWater photolysis: The formation of CH4is increased by light.d[Fe(H2O)6]3+photolysis: Under acidic conditions, light-driven CH4formation is enhanced by [Fe(H2O)6]3+photochemistry. All experiments were conducted in closed glass vials containing buffered solutions (pH 7 or pH 3) supplemented with DMSO and Fe2+or Fe3+at 30 °C (b,c) under a N2or air atmosphere. Statistical analysis was performed using paired two-tailedttests, ***p≤ 0.001. The bars are the mean + standard deviation of triplicates, shown as circles.aWas created with BioRender.com. Methane is a potent greenhouse gas, which likely enabled the evolution of life by keeping the early Earth warm. Here, we demonstrate routes towards abiotic methane and ethane formation under early-earth conditions from methylated sulfur and nitrogen compounds with prebiotic origin. These compounds are demethylated in Fenton reactions governed by ferrous iron and reactive oxygen species (ROS) produced by light and heat in aqueous environments. After the emergence of life, this phenomenon would have greatly intensified in the anoxic Archean by providing methylated sulfur and nitrogen substrates. This ROS-driven Fenton chemistry can occur delocalized from serpentinization across Earth’s humid realm and thereby substantially differs from previously suggested methane formation routes that are spatially restricted. Here, we report that Fenton reactions driven by light and heat release methane and ethane and might have shaped the chemical evolution of the atmosphere prior to the origin of life and beyond. Methane (CH 4 ) is a potent greenhouse gas which has in the past and is still today contributing to climate change [1] . Atmospherically accumulated CH 4 and ethane (C 2 H 6 ) might also explain the “faint young sun paradox”, which describes the apparent contradiction of a fainter sun (70 – 83% of the current solar energy output) but a climate that was at least as warm as today during early Earth (4.5–2.5 Ga ago) [2] , [3] , [4] . Although these CH 4 levels would be essential to keep the Earth a liquid hydrosphere to allow the evolution of life during the Archean (4.0–2.5 Ga), the source of CH 4 prior to the origin of life is still under debate [5] . While CH 4 was released by submarine volcanism, most CH 4 is suggested to be formed as side product of serpentinization [5] . After the evolution of microbial methanogenesis latest by 3.5 Ga [6] , methanogenesis could have been responsible for a CH 4 flux comparable to today [7] . Thus, methanogenesis is expected to be the main source of CH 4 during the Archean, supported by light carbon isotope values in sedimentary deposits [8] . However, isotope signals can only manifest upon reoxidation and CH 4 itself does not leave much of a signature in the geological record. Thus, the actual CH 4 concentrations and the potential abiotic sources during early Earth remain elusive. Based on mass-independent fractionation of sulfur, at least 20 ppmv CH 4 was present around 2.4 Ga ago [9] . A more recent study analyzing the fractionation of xenon isotopes suggests CH 4 levels of >5000 ppmv around 3.5 Ga ago [10] . Catling et al. expect even higher CH 4 levels at the beginning of the Archean (4 Ga) [3] before methanogenesis evolved. Yet, the processes responsible for these high CH 4 levels and their relative contributions remain controversial. Recently, we discovered a non-enzymatic CH 4 formation mechanism expected to occur in all living organisms [11] . The mechanism has been demonstrated to be active in over 30 very diverse organisms [11] and suggested to explain previously observed CH 4 formation by cyanobacteria [12] , freshwater and marine algae [13] , [14] , saprotrophic fungi [15] and plants [16] . The CH 4 formation is driven by a cascade of radical reactions, governed by the interplay of reactive oxygen species (ROS) and ferrous iron (Fe 2+ ), methylated sulfur (S)- and nitrogen (N)-compounds are oxidatively demethylated by hydroxyl radicals (∙OH) and oxo-iron(IV) complexes ([Fe IV =O] 2+ ) to yield methyl radicals (·CH 3 ) [11] . Here we show that this abiotic mechanism occurs also outside living cells and might have contributed to CH 4 levels before life emerged. All needed components: (i) methylated S- and N-compounds, (ii) Fe 2+ and (iii) ROS are found under early-earth conditions. (i) In a prebiotic world, methylated S-compounds like methanethiol, dimethyl sulfide (DMS) or dimethyl sulfoxide (DMSO) were formed abiotically under the reducing conditions of hydrothermal vents [17] , [18] , [19] or transported to Earth by carbonaceous meteorites during early Earth meteorite bombardment [20] , [21] . Upon the emergence of life, more methylated S-/N-compounds were produced by cells and organisms, i.e. methionine, dimethylsulfoniopropionate or trimethylamine [22] . (ii) Under the anoxic conditions of the early Earth, oceans were rather ferruginous, i.e. rich in Fe 2+ required for Fenton chemistry [23] , [24] , nonetheless ferric iron (Fe 3+ ) also occurred in Archean seawater [25] . Additionally, the mechanism driven by Fe 2+ can be enhanced by Fenton-promoting Fe 2+ -chelators, e.g. ATP or citrate [26] . Under anoxic conditions, Fe(III)-carboxylate complexes are photochemically reduced via ligand-to-metal charge transfer (LMCT) [27] , resulting in Fe 2+ and organic radicals [28] . (iii) Under ambient temperatures, low ROS levels exist in water that increase with heat [29] , or can be generated by photolysis or radiolysis [30] , [31] , [32] , [33] . Under acidic conditions, i.e. in volcanic lakes [34] , illumination of Fe(III)-aqua complexes ([Fe(H 2 O) 6 ] 3+ ) forms Fe 2+ and ROS [35] , [36] . Thus, we hypothesized that the Fenton reaction of Fe 2+ with H 2 O 2 , generated by heat and light, could have driven the formation of CH 4 from methylated S-/N-compounds independent of temperatures and pressures occurring at hydrothermal vents but at ambient conditions as early as the prebiotic world of the Hadean (4.5–4.0 Ga, Fig. 1a ). To identify critical components of such a mechanism, we used aqueous model systems to determine the influence of heat, light, and (bio)molecules on CH 4 formation in abiotic and biotic environments. Fig. 1: Heat and light drive CH 4 formation under abiotic conditions. a Reduced, methylated S-/N-compounds are formed abiotically in hydrothermal vents or transported to Earth by carbonaceous meteorites. Under anoxic conditions, H 2 O 2 is formed by thermolysis and photolysis of water and [Fe(H 2 O) 6 ] 3+ complexes, reacting with dissolved ferrous iron (Fe 2+ ) to hydroxyl radicals (∙OH) and [Fe IV = O] 2+ compounds that drive the oxidative demethylation of methylated S-/N-compounds, thereby facilitating CH 4 and C 2 H 6 formation. b Thermolysis: CH 4 is formed from DMSO under high temperatures. c Water photolysis: The formation of CH 4 is increased by light. d [Fe(H 2 O) 6 ] 3+ photolysis: Under acidic conditions, light-driven CH 4 formation is enhanced by [Fe(H 2 O) 6 ] 3+ photochemistry. All experiments were conducted in closed glass vials containing buffered solutions (pH 7 or pH 3) supplemented with DMSO and Fe 2+ or Fe 3+ at 30 °C ( b , c ) under a N 2 or air atmosphere. Statistical analysis was performed using paired two-tailed t tests, *** p ≤ 0.001. The bars are the mean + standard deviation of triplicates, shown as circles. a Was created with BioRender.com. Full size image Methane is formed under abiotic conditions To investigate CH 4 formation under abiotic conditions (Fig. 1a ), we designed a chemical model system consisting of a nitrogen atmosphere, a potassium phosphate-buffered solution (pH 7, expected during the Archean at 4.0 Ga [37] ) supplemented with Fe 2+ and the abiotically formed DMSO which serves as methyl donor for ROS-driven CH 4 formation. Over the course of the experiments, no pH change was observed, while low amounts of Fe(OH) 2 precipitated. In this model system, CH 4 was consistently formed from DMSO in the dark (Fig. 1b ). CH 4 formation rates increased with rising temperatures from 30 to 97 °C, consistent with the previously reported temperature-dependency of ROS levels in water [29] . While only marginal CH 4 formation rates derived from DMSO were observed at 30 °C (~0.02 μM h −1 ), rates increased 41-fold to ~0.82 μM h −1 at 97 °C. In addition, low C 2 H 6 amounts were formed (Supplementary Fig. 1 ), most likely resulting from the recombination of two methyl radicals [23] . At 37 °C, the CH 4 :C 2 H 6 ratio was ~110, with an increasing trend towards higher temperatures. As the ROS-driven CH 4 :C 2 H 6 ratios are substantially lower than those observed for archaeal methanogenesis [38] , the CH 4 :C 2 H 6 ratios could serve as indicator to distinguish microbial from abiotic processes. Light enhanced the abiotic CH 4 formation rates (Fig. 1c ) by photolysis of water and generation of H 2 O 2 at 30 °C (Supplementary Fig. 2 ). 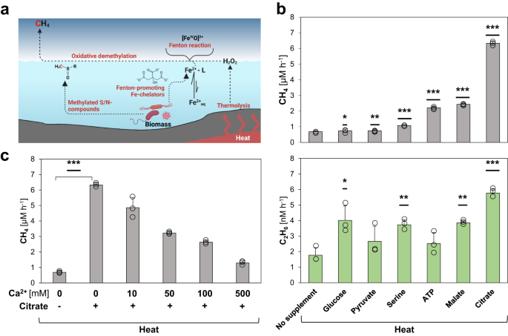Fig. 2: (Bio)molecules enhance heat-driven CH4formation. aOverview of CH4formation driven by heat. Living organisms produce S-/N-methylated compounds that serve as substrates for CH4formation and Fe2+-chelators that promote Fenton chemistry and enhance CH4formation.bHeat-driven CH4(upper panel) and C2H6(lower panel) formation is enhanced upon supplementation with (bio)molecules.cCitrate enhances heat-driven CH4formation acting as iron-chelator. Upon the addition of Ca2+, CH4levels decrease due to the replacement of Fenton-promoting Fe2+-citrate complexes with Ca2+-citrate complexes. All experiments were conducted in closed glass vials containing a buffered solution (pH 7) supplemented with DMSO, Fe2+and, optionally, citrate and Ca2+under a pure nitrogen atmosphere at 97 °C (heat). Statistical analysis was performed using paired two-tailedttests, *p≤ 0.05, **p≤ 0.01, ***p≤ 0.001. The bars are the mean + standard deviation of triplicates, shown as circles.aWas created with BioRender.com. Notably, CH 4 amounts increased ~4-fold from ~0.02 μM h −1 to ~0.08 μM h −1 upon broad-spectrum illumination (~ 350 nm < λ < ~1010 nm at 82 ± 4 µmol photons m −2 s −1 , Supplementary Fig. 3 ). This data provides evidence that light-driven CH 4 formation from methylated S-compounds can occur even in the absence of biomolecules. The addition of oxygen to the samples stopped the formation of CH 4 in this pH-neutral model system supplemented with Fe 3+ (Fig. 1c ). In contrast, under acidic (pH 3), illuminated conditions CH 4 formation rates increased ~5-fold upon Fe 3+ -supplementation in comparison to Fe 2+ -addition, indicating light-driven ROS and Fe 2+ formation from [Fe(H 2 O) 6 ] 3+ complexes (Fig. 1d ) [35] . Upon supplementation of 1 mM Fe 3+ and 1 mM Fe 2+ , keeping the overall iron concentration unchanged at 2 mM, CH 4 formation rates increased to ~0.33 μM h −1 . This 5-fold rate increase is driven by both ROS-inducing Fe 3+ and Fenton-driving Fe 2+ . Under pH-neutral conditions, mixing Fe 2+ and Fe 3+ only increased CH 4 formation rates by ~1.3-fold in comparison to Fe 2+ -supplemented samples, while only trace amounts of CH 4 were obtained from Fe 3+ -supplemented samples (Supplementary Fig. 4 ). Thus, illuminated [Fe(H 2 O) 6 ] 3+ complexes generate both Fe 2+ and ROS, thereby contributing to the ROS-driven CH 4 formation under acidic conditions. Taken together, we demonstrated that heat and light drive the formation of CH 4 and C 2 H 6 in an anoxic, abiotic environment under ambient temperatures and pressures. These results establish a ROS-driven mechanism based on Fenton chemistry that can occur delocalized from serpentinization across Earth’s humid realm and thereby substantially differs from previously suggested mechanisms that are spatially restricted. Thus, this non-enzymatic hydrocarbon formation mechanism could have released CH 4 and C 2 H 6 into the atmosphere of the Hadean and Archean. Besides CH 4 , C 2 H 6 is considered an important factor in keeping the early Earth warm, since C 2 H 6 absorbs from 11 to 13 µm in an atmospheric window (roughly 8–13 µm) where H 2 O and CO 2 do not absorb strongly [2] . Together, the hydrocarbons produced by these pathways might offer a solution to the “faint young sun paradox” [3] , [4] . (Bio)molecules enhance the heat-driven CH 4 formation Even before life emerged, several metabolites, e.g. citrate and malate, could have been formed via an ancient, non-enzymatic TCA cycle predecessor driven by ROS [39] , [40] . Catalyzed by iron particles, the formation of pyruvate from CO 2 was recently reported [41] . Intriguingly, citrate and malate, as well as other primordial (bio)molecules with a putative prebiotic origin, including ATP [42] or serine [43] , have been reported to act as Fenton-promoting Fe 2+ -chelators [26] . We therefore investigated if these hydroxylated and carboxylated (bio)molecules enhance the ROS-driven CH 4 formation rates (Fig. 2a ). Fig. 2: (Bio)molecules enhance heat-driven CH 4 formation. a Overview of CH 4 formation driven by heat. Living organisms produce S-/N-methylated compounds that serve as substrates for CH 4 formation and Fe 2+ -chelators that promote Fenton chemistry and enhance CH 4 formation. b Heat-driven CH 4 (upper panel) and C 2 H 6 (lower panel) formation is enhanced upon supplementation with (bio)molecules. c Citrate enhances heat-driven CH 4 formation acting as iron-chelator. Upon the addition of Ca 2+ , CH 4 levels decrease due to the replacement of Fenton-promoting Fe 2+ -citrate complexes with Ca 2+ -citrate complexes. All experiments were conducted in closed glass vials containing a buffered solution (pH 7) supplemented with DMSO, Fe 2+ and, optionally, citrate and Ca 2+ under a pure nitrogen atmosphere at 97 °C (heat). Statistical analysis was performed using paired two-tailed t tests, * p ≤ 0.05, ** p ≤ 0.01, *** p ≤ 0.001. The bars are the mean + standard deviation of triplicates, shown as circles. a Was created with BioRender.com. Full size image Indeed, the addition of pyruvate, glucose, serine, ATP, malate or citrate to the heat-driven (97 °C) model system increased the abiotic CH 4 formation rate, e.g. more than 11-fold for citrate (Fig. 2b ). Corresponding C 2 H 6 rates significantly increased for glucose, serine, malate and citrate, resulting in CH 4 :C 2 H 6 ratios between ~190 (glucose) and ~1100 (citrate, Fig. 2b ). To test if these enhancing effects were indeed driven by Fe 2+ chelation, we supplemented the assays with the Fe 2+ -competitor Ca 2+ (Fig. 2c ). Since (bio)molecules like citrate can alternatively chelate Ca 2+ ions, we expected that increasing Ca 2+ concentrations result in decreasing CH 4 formation rates by replacing Fenton-promoting Fe 2+ -citrate complexes with Ca 2+ -citrate complexes. Upon addition of 10 mM and 500 mM Ca 2+ , CH 4 formation rates significantly decreased from ~6.32 μM h −1 to ~4.86 μM h −1 and ~1.29 μM h −1 , respectively. Thus, 500 mM Ca 2+ suppressed ~90% of the Fenton-promoting effect of citrate supplementation. The Ca 2+ concentration-dependent decrease of the heat-driven CH 4 formation rate supports the role of citrate as a Fenton-promoting Fe 2+ -chelator, which is further indicated by citrate dissolving any ferruginous precipitate. Together, ROS generated by heat interact with iron and thereby drive the formation of methyl radicals from S-/N-methylated compounds, resulting in CH 4 and C 2 H 6 . Moreover, several hydroxylated or carboxylated (bio)molecules with a putative prebiotic origin were shown to act as Fenton-promoting Fe 2+ -chelators, indicating that ROS-driven CH 4 formation may have already been widespread within the timeframe of the transition from prebiotic chemistry to the origin of life. The rise of life would have fostered the abiotic, non-enzymatic CH 4 formation due to the consequential formation and release of biomolecules serving as chelators and substrates. A light-driven iron redox cycle sustains CH 4 formation During Fenton chemistry, Fe 2+ is either oxidized to [Fe IV = O] 2+ or ferric iron (Fe 3+ ). As Fe 3+ cannot drive Fenton reactions [23] , [24] , CH 4 formation rates decrease with increasing reaction time and increasing concentrations of Fe 3+ . While this effect may have been minor in the ferruginous Archean oceans, Fe 3+ likely dominated the iron pool in the photic zone of the oceans latest by the rise of photoferrotrophy and was also prevalent in several ecological niches, e.g. volcanic lakes [34] . The evolution of photosynthesis and the subsequent biological production of O 2 oxidized the majority of the available Fe 2+ to Fe 3+ . Thus, abiotic ROS-driven CH 4 formation would have been hindered in the sunlit realm by the late Archean in the absence of an iron redox cycle at neutral pH. Intriguingly, besides acting as Fenton-promoting Fe 2+ -chelators [26] , (bio)molecules like citrate were reported to reduce Fe 3+ to Fe 2+ via LMCT under oxic and anoxic conditions [27] . Therefore, (bio)molecules may have facilitated widespread iron redox cycling, e.g. by forming Fe(III)-carboxylate complexes. 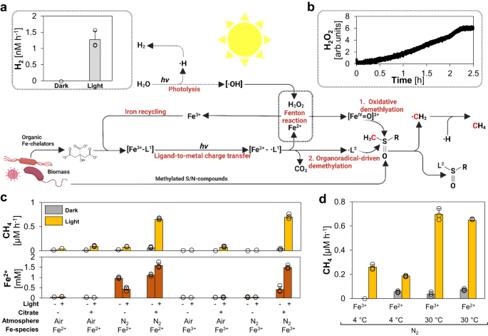Fig. 3: A light-driven iron redox cycle drives and enhances CH4formation. Upon illumination, water is photolytically split into hydroxyl radicals (·OH) and hydrogen forming H2and H2O2. Organic Fe3+-complexes (Fe3+-[L1]) are converted into Fe2+and organic radicals (·L1) via ligand-to-metal charge transfer (LMCT). The generated Fe2+reacts with H2O2to ·OH or [FeIV= O]2+and thereby drives the generation of methyl radicals (·CH3) from S-/N-methylated compounds. The LMCT-generated ·L1decomposes into CO2and another organic radical (·L2) that additionally facilitates CH4formation upon reacting with S-/N-methylated compounds. Under light, (a) H2(gray bars) and (b) H2O2is formed in pure buffer.cUpon illumination, CH4formation rates (yellow bars) are increased. Fe2+formation (brown bars) depends on anoxic conditions and is driven by LMCT induced by the addition of citrate.dLight and heat have synergistic effects on CH4formation. While heat drives CH4formation upon Fe2+-supplementation, light increases CH4formation upon Fe3+- and Fe2+-addition. All experiments were conducted in closed glass vials containing a buffered solution (pH 7) supplemented with DMSO, Fe2+or Fe3+, N2or air atmosphere in the presence or absence of citrate incubated under light or in the dark at 4 °C or 30 °C. The bars are the mean + standard deviation of triplicates, shown as circles.a,bWas created with BioRender.com. Furthermore, previous studies showed that, upon illumination of water hydroxyl radicals (·OH) and hydrogen atoms are generated, forming H 2 O 2 and H 2 [30] , [31] , [32] , [33] . Thus, we hypothesized that light could drive CH 4 formation in the absence of Fe 2+ by simultaneously (i) generating ROS from water and (ii) reducing Fe 3+ to Fe 2+ via LMCT, thereby recycling Fe 3+ and keeping the Fenton reaction running (Fig. 3 ). Fig. 3: A light-driven iron redox cycle drives and enhances CH 4 formation. Upon illumination, water is photolytically split into hydroxyl radicals (·OH) and hydrogen forming H 2 and H 2 O 2 . Organic Fe 3+ -complexes (Fe 3+ -[L 1 ]) are converted into Fe 2+ and organic radicals (·L 1 ) via ligand-to-metal charge transfer (LMCT). The generated Fe 2+ reacts with H 2 O 2 to ·OH or [Fe IV = O] 2+ and thereby drives the generation of methyl radicals (·CH 3 ) from S-/N-methylated compounds. The LMCT-generated ·L 1 decomposes into CO 2 and another organic radical (·L 2 ) that additionally facilitates CH 4 formation upon reacting with S-/N-methylated compounds. Under light, ( a ) H 2 (gray bars) and ( b ) H 2 O 2 is formed in pure buffer. c Upon illumination, CH 4 formation rates (yellow bars) are increased. Fe 2+ formation (brown bars) depends on anoxic conditions and is driven by LMCT induced by the addition of citrate. d Light and heat have synergistic effects on CH 4 formation. While heat drives CH 4 formation upon Fe 2+ -supplementation, light increases CH 4 formation upon Fe 3+ - and Fe 2+ -addition. All experiments were conducted in closed glass vials containing a buffered solution (pH 7) supplemented with DMSO, Fe 2+ or Fe 3+ , N 2 or air atmosphere in the presence or absence of citrate incubated under light or in the dark at 4 °C or 30 °C. The bars are the mean + standard deviation of triplicates, shown as circles. a , b Was created with BioRender.com. Full size image To verify our hypothesis, we first confirmed light-dependent ROS production in our model system in the absence of substrate, iron and organic ligands by measuring final reaction products of photolysis: H 2 and H 2 O 2 (Fig. 3a , b). We measured H 2 production at a rate of ~1.3 nM h −1 in anoxic samples under broad-spectrum illumination but not in samples kept in the dark (Fig. 3a ). A continuous formation of H 2 O 2 was measured online using microsensors, which confirmed light-dependent production dynamics in pure buffer (Fig. 3b ). Via fluorescence-based H 2 O 2 endpoint measurements, we found that both iron and DMSO reduced the H 2 O 2 concentrations. The decrease in H 2 O 2 levels can be attributed to Fenton reactions between H 2 O 2 , Fe 2+ and the radical scavenger DMSO (Supplementary Fig. 5 ). Building on this, we closely investigated the interplay of LMCT and iron photochemistry on CH 4 formation. For this purpose, we analyzed our chemical model system containing a buffered solution (pH 7), Fe 2+ or Fe 3+ , DMSO, in the presence or absence of citrate for the formation of CH 4 and the concentration of available Fe 2+ (Fig. 3c ). The influence of the following parameters on the formation of CH 4 was tested: (i) O 2 ( ~ 21% in air), (ii) oxidation state of the supplemented iron species (Fe 2+ vs . Fe 3 ), (iii) light and (iv) presence/absence of citrate. (i) CH 4 formation rates under anoxic conditions always exceeded rates under oxic conditions. (ii) Without citrate, initial Fe 2+ -supplementation was required to form significant CH 4 levels. (iii) CH 4 formation always increased with light. (iv) Upon citrate addition, CH 4 formation was enhanced in illuminated and anoxic samples containing DMSO and Fe 2+ or Fe 3+ . Besides elevated CH 4 formation rates, citrate addition also increased the final Fe 2+ concentrations, e.g. from ~0 mM Fe 2+ to ~1.5 mM Fe 2+ in illuminated and anoxic samples. After determining the influence of the four parameters (i) O 2 , (ii) iron (iii) light and (iv) (bio)molecules, we further investigated them individually to gain a better understanding of their contribution and role in the light-driven CH 4 formation. (i) O 2 : The influence of O 2 on LMCT and CH 4 formation was studied in citrate-supplemented samples by adding various amounts of air. Fe 2+ concentrations and CH 4 formation rates decreased with increasing O 2 levels (Supplementary Fig. 6 ). In comparison to 0 % O 2 , the Fe 2+ concentration dropped drastically already at 0.2 % O 2 and was ~96 % lower at 2 % O 2 , while CH 4 formation rates decreased approximately linearly with the O 2 level. This indicates the presence of a Fe-cycle, in which most LMCT-formed Fe 2+ is instantly re-oxidized, either by O 2 or Fenton reactions. The balance between these Fe 2+ sinks depend on O 2 availability and governs CH 4 formation rates. In the presence of O 2 , we also detected methanol (CH 3 OH) formation rates ranging from ~0.003 μM h −1 (0.2 % O 2 ) to ~0.07 μM h −1 (21 % O 2 ). CH 3 OH is preferentially formed through the reaction of ·CH 3 with O 2 [23] , [44] . Without the addition of O 2 , no CH 3 OH was detected, indicating anoxic conditions in our standard assays. (ii) Iron: The role of the LMCT-rate and the corresponding Fe 2+ availability for CH 4 formation was tested by supplementing the assays with various Fe 3+ concentrations (Supplementary Fig. 7 ). At lower Fe 3+ concentrations, CH 4 formation rates increased steeper than the measured Fe 2+ concentrations. At high Fe 3+ concentrations, CH 4 formation rates leveled off, while Fe 2+ concentrations continued to increase. This indicates that Fe 2+ is limiting the demethylation rates at low iron concentrations, because it is immediately re-oxidized, while light-dependent ROS production is limiting CH 4 formation at high iron concentrations. Most importantly, these data highlight that a light- and ROS-driven iron cycle can facilitate high rates of CH 4 formation, even in the presence of O 2 and the absence of detectable Fe 2+ , which opens the possibility of widespread abiotic CH 4 production after the great oxidation event as well as in diverse modern habitats. Next, we investigated the role of the alkali metal magnesium (Mg 2+ ) due to its high environmental abundance and found that Mg 2+ does not facilitate CH 4 formation in illuminated buffer containing DMSO and citrate (Supplementary Fig. 8 ). Upon additional Fe 3+ supplementation, Mg 2+ also decreased CH 4 formation rates by replacing Fenton-promoting Fe 3+ -citrate complexes by Mg 2+ -citrate complexes, thereby acting similar to Ca 2+ that was demonstrated to decrease heat-driven CH 4 formation (Fig. 2c ). Besides iron, the transition metals copper, cerium, cobalt, nickel and manganese were reported to drive Fenton chemistry [45] , [46] , resulting in the release of CH 4 . Thus, we tested different transition metals in our chemical model system, containing DMSO as substrate and ascorbate as a strong metal reductant [47] , [48] . We observed that copper, cobalt and cerium also enhanced CH 4 formation rates (Fig. 4a ). However, the activity of copper, cobalt and cerium was lower than iron. The high activity of iron combined with its ubiquitous abundance in the Precambrian highlights the global distribution and importance of this mechanism. Fig. 4: Transition metals, wavelengths and methylated sulfur- and nitrogen compounds mediate light-driven CH 4 formation. a Iron, cobalt and cerium enhance light-driven CH 4 formation. No significant CH 4 increase was observed for cobalt, nickel and manganese supplementation. b Light-driven CH 4 formation and Fe 2+ generation increases in the near-UV spectrum. c Light-driven formation of CH 4 from methylated S-/N-compounds (logarithmic scale). Upon illumination, significant increases in CH 4 levels were measured for dimethyl sulfide, methionine, 2-methylthioethanol, trimethylamine N-oxide and dimethyl sulfoxide (DMSO). All experiments were conducted in closed glass vials containing a buffered solution (pH 7), N 2 and either Fe 3+ or other transition metals ( a ), DMSO or other substrates ( c ) and either ascorbate ( a ) or citrate ( b , c ). Samples were incubated under broad-spectrum light ( a , c ), specific wavelengths ( b ) or in the dark at 30 °C. The dashed red line depicts the average CH 4 amounts obtained from samples illuminated by a broad-spectrum light source. Statistical analysis was performed using paired two-tailed t tests, * p ≤ 0.05, ** p ≤ 0.01, *** p ≤ 0.001. The bars are the mean + standard deviation of triplicates, shown as circles. Full size image (iii) Light: It is established that light quality has an important influence on photolysis. Short wavelength light in the ultraviolet spectrum was reported to drive water photolysis and LMCT more efficiently than longer wavelengths [49] . We expected that shorter wavelength light would increase both CH 4 formation rates and Fe 2+ levels. Indeed, CH 4 formation rates surged from ~0.3 μM h −1 (λ max = 534 nm) to ~1.23 μM h −1 (λ max = 388 nm, Fig. 4b ) and Fe 2+ concentrations almost tripled from ~1.3 mM (λ max = 534 nm) to ~4.2 mM (λ max = 388 nm). Although the broad-spectrum light had a 1.5-fold higher energy flux (57 ± 2 kJ m −2 h −1 ) compared to the 388 nm-LED light (37 ± 2 kJ m −2 h −1 ), the CH 4 formation rate under the broad-spectrum light was only half (0.7 μM h −1 ). Given that the stratospheric ozone layer was absent during the Hadean and Archaean, higher fluxes of short wavelength light ( i.e . ultraviolet light), reached aqueous environments and may have further enhanced the ROS-driven CH 4 formation. (iv) (Bio)molecules: After illumination of Fe 3+ -ligand complexes, one electron is transferred via LMCT from a carboxylated ligand (L 1 ) to Fe 3+ , an organic radical (·L 1 ), i.e. citrate radical, is generated. As described in the literature 28 , we observed the subsequent CO 2 disassembly from citrate radicals (Supplementary Fig. 9 ). We speculated that the remaining organic radical (·L 2 ) could react with DMSO, resulting in ·CH 3 and the formation of CH 4 (Fig. 3 ). Since we cannot directly detect organic radicals, we mimicked the proposed reaction in an anoxic model system only containing DMSO and the radical-generating 2,2’-azobis(2-amidinopropane) dihydrochloride (APPH) that readily decomposes into carbon-centered organic radicals at 40 °C (Supplementary Fig. 10 ). Indeed, we observed CH 4 formation in a mixture of DMSO and APPH, while only trace amounts of CH 4 were observed from either DMSO or AAPH alone, suggesting an organic radical-driven CH 4 formation mechanism. In short, carboxylates like citrate facilitate LMCT, thereby reducing Fe 3+ to Fe 2+ and forming organic radicals. Both resulting compounds drive CH 4 formation. Overall, CH 4 can be formed under anoxic conditions via (i) water thermolysis, (ii) water photolysis, (iii) [Fe(H 2 O) 6 ] 3+ photolysis and (iv) LMCT-induced carbon-centered radicals. Apart from serving as chelators, some (bio)molecules could also serve as substrates for Fenton reactions. Thus, we investigated four S-/N-methylated compounds in the presence of the chelator citrate. Upon illumination, CH 4 was formed from dimethyl sulfide, methionine, 2-methylthioethanol and trimethylamine (Fig. 4c ). These observations indicate that ROS-driven CH 4 formation significantly increased after the origin of life by providing biomolecules as chelators and substrates. Finally, synergistic effects between light and heat were observed (Fig. 3d ). For Fe 2+ -supplemented samples, CH 4 rates at 4 °C increased from ~0.056 μM h −1 in the dark over ~0.19 μM h −1 under light to ~0.65 μM h −1 in illuminated samples at 30 °C. For Fe 3+ -supplemented samples, only CH 4 rates below 0.03 μM h −1 were obtained in the dark, while CH 4 formation rates were slightly above Fe 2+ -supplemented samples in the light, again demonstrating the effects of LMCT and LMCT-induced carbon-centered radicals. Thus, the two factors heat and light synergistically combine for a stable and enhanced ROS and CH 4 formation. Biomass-derived CH 4 with an abiotic isotope fractionation Considering the impact of (bio)molecules on the LMCT-driven Fenton reaction, organic radical generation and the role of biomolecules as substrates, we expect the discussed mechanisms to have played and still play the most important role in the vicinity of decaying biomass. To demonstrate that CH 4 is indeed formed from dead biomass in the presence of a variety of biomolecules and not just in our well-defined model systems, we conducted deuterium labeling experiments. For this purpose, we grew the bacterium B. subtilis in Luria-Bertani medium supplemented with 10% D 2 O and inactivated the cells by sonication and freezing (see Methods). The obtained dead biomass was supplemented with Fe 3+ and ascorbate and incubated under broad-spectrum light. Around 40 fmol CH 4 h −1 mg −1 dry weight was obtained from labeled and unlabeled biomass (Fig. 5a ). In addition, stable hydrogen isotope values ( δ 2 H) of CH 4 from D 2 O-treated biomass showed strong enrichment in deuterium (~5900 ‰) in comparison to unlabeled biomass (~−225 ‰), demonstrating a direct conversion of isotopically labeled biomass to CH 4 . This suggests that the availability of biomass, upon the emergence of life, has increased the CH 4 formation by delivering both (i) S-/N-methylated compounds and (ii) Fenton-promoting iron chelators. The presence of CH 4 has been suggested to be crucial for the evolution of life, since it could serve as life´s first carbon source via methanotrophy [50] , [51] , [52] . Following this line of thought, we could demonstrate that methanotrophic Methylocystis hirsuta grew on CH 4 generated by our light-driven model system, transferred to the headspace of the M. hirsuta culture (Supplementary Fig. 11 ). In fact, the “last methane-metabolizing ancestor” had likely the genes to perform methanogenesis and anaerobic methane oxidation [53] , suggesting that, under high CH 4 concentrations, methanotrophy could have emerged prior to methanogenesis. Fig. 5: Isotope labeling studies confirm dead biomass as substrate and show an abiotic isotope fractionation for ROS-driven CH 4 formation. a Unlabeled or deuterium-enriched CH 4 is formed from unlabeled biomass (gray dots) or deuterated biomass (red dots), respectively. b Stable carbon isotope values of cultures from the methanogen Methanothermobacter marburgensis , heat-, or light-generated CH 4 . All experiments were conducted in closed glass vials containing a buffered solution ( a , b —heat, light) or culture medium ( b —methanogenesis), supplemented with Fe 3+ and ascorbate ( a ) or Fe 2+ and citrate ( b —heat, light) under a nitrogen atmosphere, incubated under light at 30 °C or in the dark at 97 °C. Statistical analysis was performed using paired two-tailed t tests, * p ≤ 0.05. The bars are the mean + standard deviation of triplicates, shown as circles. Full size image Finally, we speculated that ROS-driven CH 4 formation leads to different stable carbon isotope values ( δ 13 C ) compared to biological processes, i.e ., methanogenesis. The observed δ 13 C values for CH 4 generated by heat or light were less negative (~−54 ± 1.1‰) compared to the δ 13 C value of the methanogen Methanothermobacter marburgensis (~−59.2 ± 2.3‰, Fig. 5b ). While the isotopic fractionation during abiotic ROS-driven CH 4 formation remains to be studied in depth, these results suggest a lower carbon isotope fractionation for ROS-driven CH 4 formation than for enzymatic methanogenesis. Together with the observed CH 4 :C 2 H 6 ratios, isotopic signatures may therefore serve to differentiate between CH 4 formed enzymatically or abiotically on Earth and extraterrestrial planets. In this work, we demonstrated that the interplay of Fe 2+ and H 2 O 2 , generated by heat and light, drives CH 4 and C 2 H 6 formation from methylated S-/N-compounds via Fenton chemistry under conditions that were globally prevalent in the Hadean and Archean. As we observed CH 4 formation under suboxic and oxic conditions, these mechanisms could, in principle, also contribute to extant CH 4 emissions from aqueous environments that were recently shown to correlate with light instead of specific enzymatic pathways [54] . The here described pathways allow CH 4 and C 2 H 6 formation in many aqueous environments including oceans, lakes, rivers, and ponds, delocalized from restricted hotspots for (bio)molecule formation such as hydrothermal vents or ultramafic rocks, in superficial water layers driven by light and throughout the entire water column driven by heat. After the emergence of life, this phenomenon would have greatly intensified in the anoxic Archaean and the subsequent “boring billion” [55] , [56] . The increasing amounts of biomass provided methylated S-/N-substrates, Fe-chelating biomolecules reducing Fe 3+ to Fe 2+ and releasing organic radicals and thus enhance ROS-driven CH 4 formation. Possibly, these reactions facilitated elevated CH 4 and C 2 H 6 levels during the Hadean and Archean. These hydrocarbons would have contributed to atmospheric temperatures on Earth and allowed the evolution of life in a liquid hydrosphere which could have influenced the evolution of metabolism by allowing the rise of methanotrophy prior to methanogenesis. This work lays the foundation to explore further the mechanism’s role in shaping the evolution of the atmosphere on Earth and other planets and its influence on the current climate change. General assay conditions Unless otherwise indicated, 4 mL samples were incubated in closed 20 mL glass vials at 30 °C under a pure nitrogen (N 2 ) atmosphere and subsequently analyzed via gas chromatography (GC). Heat assays In total, 500 mM DMSO and 10 mM FeSO 4 were added to 20 mM degassed potassium phosphate buffer (pH 7) in an anaerobic tent. The headspace of the closed vials was then cycled three times with vacuum and N 2 . Samples were incubated at 37 °C, 57 °C, 77 °C and 97 °C for 6 h in an incubator in the dark. Optionally, 20 mM citrate, malate, ATP, serine, glucose or pyruvate were also supplemented. Ca 2+ was added in the form of CaCl 2 . Samples were measured within the linear range of CH 4 formation rate via gas chromatography. Light assays In total, 500 mM DMSO, 2 mM of either FeCl 3 or FeSO 4 and, optionally, 10 mM citrate were added to 20 mM degassed potassium phosphate buffer (pH 7). Anoxic conditions were generated by drawing vacuum eight times for 1 min and a subsequent filling with N 2 . For experiments investigating [Fe(H 2 O) 6 ] 3+ complexes, samples were incubated under anoxic, acidic conditions (20 mM Tris · HCl buffer, pH 3) and supplemented with 500 mM DMSO and either 2 mM FeCl 3 , 2 mM FeSO 4 or 1 mM FeCl 3 and 1 mM FeSO 4 , each. For the investigation of transition metals (Fig. 4a ), 2 mM cerium (CeNH 4 SO 4 ), manganese (MnSO 4 ), cobalt (CoNO 3 ), nickel (NiSO 4 ), copper (CuCl 2 ) or iron (FeCl 3 ) and 10 mM pH-neutral ascorbate were added to 500 mM DMSO and 20 mM potassium phosphate buffer with an incubation for 1 day. The effect of different wavelengths on CH 4 formation (Fig. 4b ) was investigated by adding 5 mM FeCl 3 , 10 mM citrate and 500 mM DMSO to 20 mM potassium phosphate buffer with an incubation for 1 day. For the determination of substrates for CH 4 formation (Fig. 4c ), 500 mM DMS, methionine, 2-methylthioethanol, Trimethylamine N-oxide or DMSO were added to 10 mM FeCl 3 and 100 mM citrate in 20 mM potassium phosphate buffer with an incubation for 3 days. Samples were incubated under air or N 2 in the dark or under constant broad-spectrum illumination from light bulbs (Osram, Superlux, Super E SIL 60; Φ = 82 ± 4 µmol photons m −2 s −1 , H = 52 ± 2 kJ m −2 h −1 ; Supplementary Fig. 3 ) for 1 day. Samples were measured within the linear range of the CH 4 formation via gas chromatography. Specific wavelengths were provided by diodes (H2A1 series, Roithner Lasertechnik, Austria) emitting UV-A, blue, cyan, green, red or near-infrared light (λ max = 388 nm, Φ = 35 ± 1 µmol photons m −2 s −1 , H = 36 ± 2 kJ m −2 h −1 ; λ max = 436 nm, Φ = 45 ± 1 µmol photons m −2 s −1 , H = 45 ± 1 kJ m −2 h −1 ; λ max = 500 nm, Φ = 64 ± 4 µmol photons m −2 s −1 , H = 55 ± 3 kJ m −2 h −1 ; λ max = 534 nm, Φ = 63 ± 1 µmol photons m −2 s −1 , H = 50 ± 1 kJ m −2 h −1 ; λ max = 675 nm, Φ = 45 ± 4 µmol photons m −2 s −1 , H = 29 ± 3 kJ m −2 h −1 ; or λ max = 868 nm, Φ = 69 ± 7 µmol photons m −2 s −1 , H = 35 ± 3 kJ m −2 h −1 ) Light intensity was determined using a fiber optic scalar irradiance microsensor [57] connected to a spectrometer (USB4000; Ocean Optics, USA) placed in the center of the incubation vials and calibrated using a spherical light probe (Walz) connected to a LI-250A light meter (Li-Cor Biosciences GmbH, Germany) [58] . 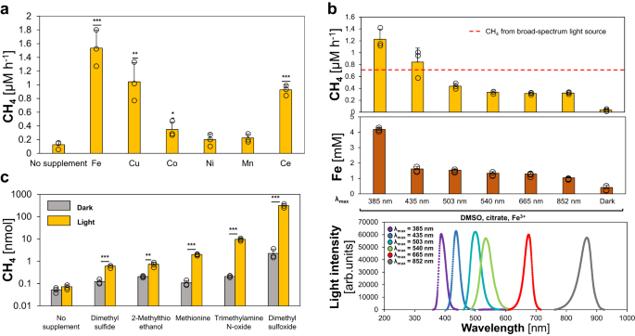Fig. 4: Transition metals, wavelengths and methylated sulfur- and nitrogen compounds mediate light-driven CH4formation. aIron, cobalt and cerium enhance light-driven CH4formation. No significant CH4increase was observed for cobalt, nickel and manganese supplementation.bLight-driven CH4formation and Fe2+generation increases in the near-UV spectrum.cLight-driven formation of CH4from methylated S-/N-compounds (logarithmic scale). Upon illumination, significant increases in CH4levels were measured for dimethyl sulfide, methionine, 2-methylthioethanol, trimethylamine N-oxide and dimethyl sulfoxide (DMSO). All experiments were conducted in closed glass vials containing a buffered solution (pH 7), N2and either Fe3+or other transition metals (a), DMSO or other substrates (c) and either ascorbate (a) or citrate (b,c). Samples were incubated under broad-spectrum light (a,c), specific wavelengths (b) or in the dark at 30 °C. The dashed red line depicts the average CH4amounts obtained from samples illuminated by a broad-spectrum light source. Statistical analysis was performed using paired two-tailedttests, *p≤ 0.05, **p≤ 0.01, ***p≤ 0.001. The bars are the mean + standard deviation of triplicates, shown as circles. 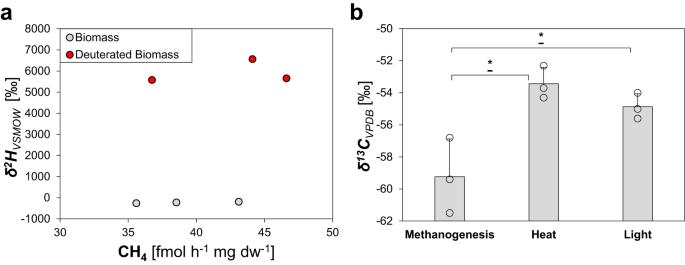Fig. 5: Isotope labeling studies confirm dead biomass as substrate and show an abiotic isotope fractionation for ROS-driven CH4formation. aUnlabeled or deuterium-enriched CH4is formed from unlabeled biomass (gray dots) or deuterated biomass (red dots), respectively.bStable carbon isotope values of cultures from the methanogenMethanothermobacter marburgensis, heat-, or light-generated CH4. All experiments were conducted in closed glass vials containing a buffered solution (a,b—heat, light) or culture medium (b—methanogenesis), supplemented with Fe3+and ascorbate (a) or Fe2+and citrate (b—heat, light) under a nitrogen atmosphere, incubated under light at 30 °C or in the dark at 97 °C. Statistical analysis was performed using paired two-tailedttests, *p≤ 0.05. The bars are the mean + standard deviation of triplicates, shown as circles. Concentration of Fe 2+ was quantified with the colorimetric ferrozine method [59] . Bacillus subtilis biomass assays B. subtilis was grown in 500 mL LB media, supplemented with 10 % H 2 O or D 2 O, grown for 36 h at 37 °C and 180 rpm. The obtained culture was collected by three cycles of centrifugation (10 min, 4743 × g ) and resuspended in 35 mL 20 mM potassium phosphate buffer (pH 7) in order to remove the excess D 2 O. Biomass was then generated by sonication (4-times, 1 min) and freezing of the samples. Subsequently, 80 mL buffer was supplemented with 10 mL biomass, 20 mM FeCl 3 and 50 mM ascorbic acid, saturated with N 2 for 30 min and incubated in 100 mL closed glass vials under N 2 and constant broad-spectrum illumination for 3 days. The gas headspace was extracted with a syringe and analyzed with regard to CH 4 content and δ 2 H values. Methylocystis hirsuta and Methanothermobacter marburgensis cultivation M. hirsuta growth media contained 0.5 g Na 2 HPO 4 · 2H 2 O, 0.22 g KH 2 PO 4 , 1 g KNO 3 , 0.4 mg CaCl 2 · 2H 2 O, 2 mg MgSO 4 · 7H 2 O per liter, supplemented with 5 mg Na 2 EDTA, 0.06 mg CuCl 2 · 5H 2 O, 2 mg FeSO 4 · 7H 2 O, 0.1 mg ZnSO 4 · 7H 2 O, 0.03 mg MnCl 4 · 4H 2 O, 0.05 mg H 3 BO 3 , 0.2 mg CoCl 2 · 6H 2 O, 0.02 mg NiCl 2 · 6H 2 O and 0.03 mg Na 2 MoO 4 · 2H 2 O per liter. M. hirsuta was cultivated in 100 mL closed glass vials containing 30 mL culture and was incubated at 25 °C and 150 rpm under an air atmosphere. Methane was produced by supplementing 2 L degassed 20 mM potassium phosphate buffer with 1 M DMSO, 25 mM FeSO 4 and 50 mM ascorbic acid, incubating the solution under constant illumination in 1 L flasks and collecting the formed CH 4 with syringes. M. hirsuta cultures were either supplemented with 25 mL light-generated CH 4 or 25 mL pure N 2 . M. marburgensis was cultivated as previously described [60] . Continuous H 2 O 2 measurements using microsensors To visualize H 2 O 2 production in the illuminated anoxic model system, an H 2 O 2 microsensor was positioned in the solution. The H 2 O 2 microsensors were built, calibrated and used as described previously [61] . We sealed the vial opening with self-adhesive tape, rigorously bubbled the liquid with N 2 and then adjusted a gentle flow of N 2 through the headspace to minimize oxygen input from the atmosphere. Light was provided from halogen lamps (KL2500, Schott) at an intensity of 1027 µmol photons m −2 s −1 . We did not attempt to calculate light-dependent H 2 O 2 production rates due to the open design of the system, which allowed for the exchange of H 2 O 2 with the headspace across the water interface. End-point H 2 O 2 measurements After illumination, 290 µL sample was mixed anaerobically with 9 µL Amplex Ultrared (Thermofisher, A36006, 30 µM final concentration) and 1 µL recombinant APEX2 (0.23 µM final concentration). Fluorescence was then measured with a plate reader (BMG ClarioStar™) at 568 nm excitation / 581 nm emission. A calibration curve was established with H 2 O 2 following the same procedure. To prevent O 2 -driven H 2 O 2 generation while sample preparation, all buffers were saturated with N 2 and the plate reader was kept at a partial oxygen pressure of 0.1% with an atmospheric control unit (Clariostar, BMG). Before sample preparation, all sample components (20 mM potassium phosphate buffer, DMSO, 1 M citrate and 100 mM FeCl 3 ) were degassed and kept in an anoxic tent overnight. Quantification of CH 4 , C 2 H 6, CO 2 , and H 2 (GC-FID) Amounts of formed CH 4 , C 2 H 6 , CO 2 and H 2 were determined via headspace analysis using a PerkinElmer® Clarus®690 GC system (GC–‍FID/TCD) with a custom-made column circuit (ARNL6743). The headspace samples were injected by a TurboMatrixX110 (PerkinElmer Inc, Waltham, USA) autosampler, heating the samples to 45 °C for 15 min prior to injection. The samples were then separated on a HayeSep column (7’ HayeSep N 1/8” Sf; PerkinElmer®), followed by molecular sieve (9’ Molecular Sieve 13×1/8” Sf; PerkinElmer®) kept at 60 °C. Subsequently, the gases were detected with a flame ionization detector (FID, at 250 °C) and a thermal conductivity detector (TCD, at 200 °C). The quantification of CH 4 , C 2 H 6 , CO 2 and H 2 was based on linear standard curves that were derived from measuring varying amounts of these gases. CH 3 OH measurements (GC-FID) CH 3 OH was quantified with a GC-FID (Shimadzu GC-2010 Plus, FID-2010 Plus, 280 °C) containing an AOC 20i autosampler and a ZB-WAXplus (Zebron) column (30 m x ⌀ = 0.25 mm, df, 0.25 µm). A H 2 O sample (1 μL) was injected in the split liner (250 °C, split 5,15,50). The temperature program was kept at 35 °C for 5 min and then increased by 50 °C min −1 until 200 °C which was kept for 3 min. Helium served as carrier gas (flow rate: 1.95 ml min −1 ) and the FID was operated with 400 ml min −1 synthetic air, 40 ml min −1 H 2 and 30 ml min −1 N 2 , serving as a makeup gas. For Split 5, a calibration curve (R 2 = 0.9931) was generated by diluting CH 3 OH (99.9% purity), while an R 2 = 0.9981 for split 15 and an R 2 = 0.9997 for split 50 was determined. δ 13 C stable isotope measurements (GC-C-IRMS) δ 13 C values of CH 4 were determined by gas chromatography-combustion-isotope ratio mass spectrometry (GC-C-IRMS). Aliquots of headspace gas were transferred to an evacuated sample loop (40 mL) and a cryogenic pre-concentration unit to trap CH 4 . CH 4 was trapped on HayeSep D, separated from interfering compounds by GC and transferred to the GC-C-IRMS. The system consists of a cryogenic pre-concentration unit directly connected to an HP 6890 N GC (He flow rate: 1.8 mL min −1 ; Agilent Technologies, Santa Clara, USA) fitted with a GS-Carbonplot capillary column (30 m * 0.32 mm i.d., d f 1.5 µm; Agilent Technologies) and a PoraPlot capillary column (25 m * 0.25 mm (i.d. ), d f 8 µm; Varian, Lake Forest, USA). The GC flow was coupled using a press-fit connector to a combustion reactor comprised of an oxidation reactor (ceramic tube (Al 2 O 3 ), length 320 mm, inner diameter 0.5 mm, with oxygen-activated Cu/Ni/Pt wires inside; reactor temperature 960 °C) and a GC Combustion III Interface (ThermoQuest Finnigan) to decompose CH 4 into CO 2 . 13 C/ 12 C ratios were determined with a Delta PLUS XL mass spectrometer (ThermoQuest Finnigan, Bremen, Germany). High-purity CO 2 (Messer Griesheim, Frankfurt, Germany) was used as the working monitoring gas. 13 C/ 12 C ratios (δ 13 C values) are expressed in the conventional δ notation in per mil versus VPDB, calculated as: 
    δ^13C_VPDB=((13C/12C)_Sample/(13C/12C)_Standard)-1
 (1) δ 13 C values were corrected using three reference standards of high-purity CH 4 with δ 13 C values of –54.5 ± 0.2 ‰ (Isometric Instruments, Victoria, Canada), –66.5 ± 0.2 ‰ (Isometric Instruments) and –42.3 ± 0.2 ‰ (in-house), calibrated against International Atomic Energy Agency and NIST reference substances. δ 2 H stable isotope measurements (GC-TC-IRMS) δ 2 H values for CH 4 were determined using GC-temperature conversion-isotope ratio mass spectrometry (GC-TC-IRMS). The analytical set-up was the same as the one used for δ 13 C stable isotope measurements except that the He flow rate was changed to 0.6 ml min −1 and, instead of combustion to CO 2 and H 2 O, CH 4 was thermolytically converted (at 1450 °C) to hydrogen and carbon. After IRMS measurements, the obtained δ 2 H values were corrected by using two reference standards of high-purity CH 4 with δ 2 H values of –149.9‰  ±  0.2‰ (T-iso2, Isometric Instruments) and –190.6‰  ±  0.2‰ (in house). All δ 2 H values are expressed in the conventional δ notation in per mil versus Vienna Standard Mean Ocean Water (VSMOW), calculated as 
    δ^2H_VSMOW=((2H/1H)_Sample/(2H/1H)_Standard)-1
 (2) Statistics Unless indicated otherwise, all experiments were performed with N = 3 replicates (3 biological replicates). To test for significant differences in CH 4 formation between two samples, single-factor analysis (two-tailed students t test) of variance (ANOVA) was used.